Perinuclear tethers license telomeric DSBs for a broad kinesin- and NPC-dependent DNA repair process DNA double-strand breaks (DSBs) are often targeted to nuclear pore complexes (NPCs) for repair. How targeting is achieved and the DNA repair pathways involved in this process remain unclear. Here, we show that the kinesin-14 motor protein complex (Cik1–Kar3) cooperates with chromatin remodellers to mediate interactions between subtelomeric DSBs and the Nup84 nuclear pore complex to ensure cell survival via break-induced replication (BIR), an error-prone DNA repair process. Insertion of a DNA zip code near the subtelomeric DSB site artificially targets it to NPCs hyperactivating this repair mechanism. Kinesin-14 and Nup84 mediate BIR-dependent repair at non-telomeric DSBs whereas perinuclear telomere tethers are only required for telomeric BIR. Furthermore, kinesin-14 plays a critical role in telomerase-independent telomere maintenance. Thus, we uncover roles for kinesin and NPCs in DNA repair by BIR and reveal that perinuclear telomere anchors license subtelomeric DSBs for this error-prone DNA repair mechanism. The DNA replication machinery cannot copy the ends of linear chromosomes. To prevent this limitation from leading to the rapid erosion of chromosomes over cycles of DNA replication and cell division, the ends of linear chromosomes consist of telomeres, or repetitive DNA sequences whose length can be maintained by the enzyme telomerase [1] , [2] . In addition, telomeres act as recruitment sites for chromosomal complexes that then spread and establish silent chromatin or heterochromatin structures within neighbouring regions known as subtelomeres [3] , [4] . DNA double-strand breaks (DSBs) within heterochromatic repetitive DNA constitute a great risk to eukaryotic genome stability. In yeast, DSBs within the highly repetitive ribosomal RNA genes (rDNA) can lead to unequal sister chromatid exchange events, compromise chromosome stability and shorten cellular lifespan [4] , [5] , [6] , [7] . DSBs within rDNA repeats were found to transiently exit the Rad52/recombination-repressive environment of the nucleolus in which they typically reside to undergo repair without compromising genome integrity [8] , [9] . In flies, heterochromatic DSBs exit their Rad51/recombination-repressive subnuclear domain to undergo repair [10] . Similarly, heterochromatic DSBs were found to relocate outside their domain for repair in cultured human cells [11] . Therefore, DSBs within heterochromatic repetitive DNAs can exit their nuclear domain to undergo repair. DSBs escaping their repressive nuclear environment may also be targeted to repair-promoting nuclear regions, such as specific locations along the nuclear envelope. In yeast, these locations are the nuclear pore subcomplex Nup84 (composed of seven entities, including Nup84 and Nup145) as well as the Mps3 inner nuclear membrane protein [12] , [13] , [14] , [15] . In fact, DSBs in cells without clear donor DNA sites for repair relocate at least transiently to Nup84 or Mps3 proteins [12] , [13] , [14] , [15] . All 32 telomeres of budding yeast are arranged in a handful of clusters at certain points along the nuclear envelope [16] . These telomeric clusters do not co-localize with nuclear pore complexes [17] . Intriguingly, the ability to survive a subtelomeric DSB is dependent on Nup84 as well as a number of factors known to anchor telomere clusters to the nuclear envelope [12] , [13] , [18] , [19] , [20] , [21] , [22] . However, the relationship between perinuclear telomere tethers and nuclear pore subcomplexes in subtelomeric DNA repair remains unknown [12] , [23] . In addition, it is unclear whether survival is achieved through bona fide DNA repair processes such as non-homologous end joining (NHEJ) or rather via genome patching mechanisms that may help propagate a compromised genome [24] , [25] , [26] . Moreover, how DSB sites move within the nucleus is unclear. Here, we uncover a role for the kinesin-14 motor protein complex in the transient relocation of telomeric and non-telomeric DSBs to Nup84 and reveal that this function promotes break-induced replication (BIR), a recombination-based error-prone DNA repair mechanism. Perinuclear telomere tethers such as cohibin are required for telomeric DSBs to utilize this broader DNA repair process, which also relies on the DNA damage response, chromatin remodelling, microtubules and Mps3. We also find that kinesin-14 counteracts senescence by ensuring efficient recombination-based telomere maintenance in the absence of telomerase. Overall, our work identifies specific roles for motor and nuclear envelope proteins in the promotion of a broad and error-prone DNA repair mechanism while having potentially critical implications for our understanding of genome instability-linked diseases including cancer. Genetic analysis of subtelomeric DSB repair To gain insight into the mechanisms by which DNA breaks in subtelomeric regions are repaired, we used cells in which an inducible DSB can be triggered at either a subtelomeric or a more internal control region on the left arm of chromosome XI (Chr. XI; Fig. 1a ) [22] , [27] . In both of the cases, we introduced galactose-inducible I-SceI endonuclease in cells harbouring a URA3 marker gene flanked by two inverted I-SceI cut sites, which enabled us to confirm successful DSB induction by culturing cells on selective media and monitoring for URA3 reporter loss ( Fig. 1a ; Supplementary Fig. 1 ). Deletion of the Nup84 subcomplex components Nup84 or Nup145, or of the perinuclear telomere-tethering protein Esc1, significantly decreased survival of the subtelomeric DSB, as expected ( Fig. 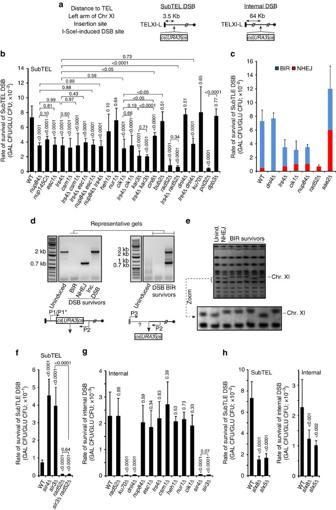Figure 1: Perinuclear and motor protein complexes ensure subtelomeric DSB survival. (a) Schematic illustrating galactose-inducible DSB site within a subtelomeric (SubTEL) and internal region of Chromosome (Chr.) XI. (b) Genetic analysis of subtelomeric DSB survival. Survival (mean±s.d.;N=5) is compiled and presented as the ratio of colony-forming units on galactose (GAL) relative to glucose (GLU). Presented immediately above mutants arePvalues (t-test) relative to wild type. OtherPvalues are as illustrated on the graph. Relative survival is inSupplementary Table 1. (c) Proportions of survivors (mean±s.d.;N=30) using BIR or NHEJ are revealed by PCR analysis using primers amplifying regions surrounding the DSB site. Error bars for overall survival rate are shown. (d,e) Representative subtelomeric DSB survivor analysis. (d) Agarose gels with corresponding primer pairs used right below showing how different PCR products amplified across the DSB site after induction/survival indicate different repair pathways. Survivors were initially analysed and categorized into BIR (no product), NHEJ (∼0.7 kb product) or incomplete DSB (∼2 kb product; very rare). All BIR survivors were subsequently analysed using a generic telomere AC1-3primer with a small fraction of survivors yielding products. All PCR products were amplified using their respective primers as illustrated (P1* used for zip/control sequence strains for initial analysis). (e) EtBr-stained CHEF gel showing changes to the size of Chr. XI in wild-type BIR survivors relative to uninduced and NHEJ survivors. (f–h) Compiled subtelomeric or internal DSB survival assays reveal that survival of a subtelomeric, but not an internal, DSB located on the left arm of Chr. XI is dependent on cohibin/Esc1, Cik1 and Nup84 proteins (mean±s.d.;N=5).Pvalues (t-test) comparing mutants to wild-type cells are immediately above bars with additional statistical comparisons as shown. (f) Disruption of telomeric SIR proteins increases Rad52-dependent survival of a subtelomeric DSB. (g) Deletion of the NHEJ factors Ku70/Dnl4 or SIR proteins, but not telomere tethers, motor proteins nor NPC components, decreases survival of an internal DSB. (h) Disruption of the Slx5–Slx8 complex compromises both subtelomeric and internal DSB survival. 1b ; Supplementary Table 1 ) [21] , [22] , [28] . Disruption of the telomere-tethering complex cohibin (composed of Lrs4 and Csm1 proteins) alone or in combination with Esc1 deletion, similarly compromised subtelomeric DSB survival ( Fig. 1b ) [6] , [8] . Combining the deletion of Nup84 with the disruption of Esc1 or cohibin did not further lower survival rates indicating that all of these factors likely operate within the same pathway ( Fig. 1b ). Importantly, heh1 Δ or nur1 Δ cells, which retain perinuclear telomere anchoring, did not exhibit significant reductions in DSB survival rates ( Fig. 1b ) [6] . Since telomere clusters do not generally co-localize with nuclear pore complexes at the nuclear periphery, we wondered whether motor proteins might target subtelomeric DSBs to the nuclear pore complexes [16] . Interestingly, genes encoding for cohibin subunits exhibit negative genetic interactions with Cik1 and Kar3, which localize to the nucleus and together constitute the kinesin-14 motor protein complex [29] , [30] , [31] , [32] , [33] , [34] , [35] . Indeed, disruption of kinesin-14 alone or in combination with Lrs4 deletion, decreased subtelomeric DSB survival to levels similar to those seen in cells deficient in cohibin or Nup84 ( Fig. 1b ). Kar3-deficient cells exhibited qualitatively greater drops in survival than cik1 Δ cells ( Fig. 1b ). This may be related to the Cik1-independent Kar3 function, which is shared with Vik1 and Cin8, at the mitotic spindle poles [36] . Consistent with this rationale, cin8 Δ cells displayed only a partial decrease in DSB survival ( Fig. 1b ). In addition, deletion of the spindle checkpoint protein Bub2 had no significant effect on DSB survival ( Fig. 1b ). More importantly, deletion of the homologous recombination factor Rad52, but not the NHEJ factors Dnl4 or Ku70, greatly decreased the subtelomeric DSB survival rates of wild-type and lrs4 Δ cells ( Fig. 1b ). Many proteins including the Ku complex (composed of Ku70 and Ku80) and telomerase contribute to a perinuclear telomere-tethering process that is somewhat distinct from cohibin-dependent tethering [13] , [20] , [37] , [38] . Since Ku disruption is ineffectual in our subtelomeric DSB survival assay ( Fig. 1b ), this points to a survival pathway that is more dependent on cohibin and Esc1 telomere tethers, at least within our experimental system. Figure 1: Perinuclear and motor protein complexes ensure subtelomeric DSB survival. ( a ) Schematic illustrating galactose-inducible DSB site within a subtelomeric (SubTEL) and internal region of Chromosome (Chr.) XI. ( b ) Genetic analysis of subtelomeric DSB survival. Survival (mean±s.d. ; N =5) is compiled and presented as the ratio of colony-forming units on galactose (GAL) relative to glucose (GLU). Presented immediately above mutants are P values ( t -test) relative to wild type. Other P values are as illustrated on the graph. Relative survival is in Supplementary Table 1 . ( c ) Proportions of survivors (mean±s.d. ; N =30) using BIR or NHEJ are revealed by PCR analysis using primers amplifying regions surrounding the DSB site. Error bars for overall survival rate are shown. ( d , e ) Representative subtelomeric DSB survivor analysis. ( d ) Agarose gels with corresponding primer pairs used right below showing how different PCR products amplified across the DSB site after induction/survival indicate different repair pathways. Survivors were initially analysed and categorized into BIR (no product), NHEJ ( ∼ 0.7 kb product) or incomplete DSB ( ∼ 2 kb product; very rare). All BIR survivors were subsequently analysed using a generic telomere AC 1-3 primer with a small fraction of survivors yielding products. All PCR products were amplified using their respective primers as illustrated (P1* used for zip/control sequence strains for initial analysis). ( e ) EtBr-stained CHEF gel showing changes to the size of Chr. XI in wild-type BIR survivors relative to uninduced and NHEJ survivors. ( f – h ) Compiled subtelomeric or internal DSB survival assays reveal that survival of a subtelomeric, but not an internal, DSB located on the left arm of Chr. XI is dependent on cohibin/Esc1, Cik1 and Nup84 proteins (mean±s.d. ; N =5). P values ( t -test) comparing mutants to wild-type cells are immediately above bars with additional statistical comparisons as shown. ( f ) Disruption of telomeric SIR proteins increases Rad52-dependent survival of a subtelomeric DSB. ( g ) Deletion of the NHEJ factors Ku70/Dnl4 or SIR proteins, but not telomere tethers, motor proteins nor NPC components, decreases survival of an internal DSB. ( h ) Disruption of the Slx5–Slx8 complex compromises both subtelomeric and internal DSB survival. Full size image As Rad52 is implicated in different DNA recombination processes, we asked whether a specific type of recombinational repair was implicated at subtelomeric DSBs. Genomic analysis of wild-type survivors by PCR as well as contour-clamped homogeneous electric field electrophoresis (CHEF) revealed that cells relied primarily on BIR, which is typically engaged when DNA sequences only on one side of the DSB have a homologous template ( Fig. 1c–e ). In contrast, only a small fraction of cells underwent Dnl4/NHEJ-dependent repair ( Fig. 1c,d ). In addition, deletion of the BIR factor DNA Polα subunit Pol32, but not control Polɛ subunit Dpb3, significantly decreased subtelomeric DSB survival to levels similar to those seen in Rad52-deficient cells ( Fig. 1b ) [39] . Moreover, disruption of Rad52, Lrs4, Cik1 or Nup84 specifically decreased BIR-dependent DSB survival ( Fig. 1c,d ). Furthermore, we found that deletion of the resection factor Sae2 increased overall DSB survival and the percentage of NHEJ-dependent survivors, consistent with the notion that resection suppresses NHEJ ( Fig. 1c ) [40] , [41] , [42] , [43] . Thus, cohibin/Esc1 perinuclear telomere tethers, kinesin-14, nuclear pore subcomplexes and DNA resection cooperate to ensure BIR-dependent repair of a subtelomeric DSB. Loss of perinuclear telomere tethering compromises SIR (silent information regulator)-dependent silent chromatin assembly but SIR deletions promoted Rad52-dependent repair, pointing to a dominant SIR-independent role for cohibin/Esc1, kinesin-14 and Nup84 in BIR-dependent subtelomeric DSB repair ( Fig. 1f ) [4] , [6] . This is also consistent with the notion that the complete loss of telomeric silencing observed in SIR-deficient cells promotes access to the DSB repair machinery. In contrast, survival of the internal DSB was greatly dependent on SIR proteins as well as the NHEJ factors Dnl4 and Ku70, but not on Rad52, telomere tethers, motor or nuclear pore proteins ( Fig. 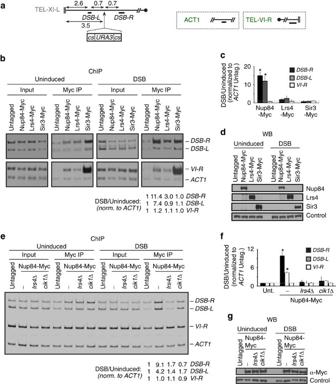Figure 2: Cohibin and kinesin-14 mediate interaction of subtelomeric DSBs with Nup84. (a) Schematic illustrating positions of PCR products used in ChIP to assess interactions between the subtelomeric DSB and various proteins. (b,c) Anti-Myc-tagged protein ChIP reveals increased interactions between the subtelomeric DSB and Nup84. Representative gels withACT1-normalized relative enrichments (b) and quantifications (c) are shown (mean±s.d.;N=3; *,t-testP<0.05). (d) Anti-Myc immunoblotting indicates that DSB induction did not alter the level of Myc-tagged proteins used in ChIP analyses. Sir3-Myc served as positive control. (e,f) Anti-Myc-tagged protein ChIP also reveals that subtelomeric DSB–Nup84 interactions require Lrs4 and Cik1. Representative gels withACT1-normalized relative enrichments (e) and quantifications (f) are shown (mean±s.d.;N=3; *,t-testP<0.05). (g) Anti-Myc immunoblotting indicates that DSB induction did not alter the level of Myc-tagged proteins used in ChIP analyses. Untag., untagged. 1g ; Supplementary Table 2 ). Deletion of Slx5/Slx8 proteins, which are linked to DNA repair both at the nuclear periphery and more internally within the nucleus, decreased survival rates in both subtelomeric and internal DSB repair assays, as expected ( Fig. 1h ) [12] . Together, our findings so far indicate that the herein studied BIR-dependent repair mechanism is different from silent chromatin assembly and does not act at a more internal DSB site that is on the same chromosome and is more dependent on NHEJ. Licensing and microtubules at remodelled subtelomeric DSBs Next, we asked whether cohibin and kinesin-14 proteins promote the physical interaction of the subtelomeric DSB with the Nup84 nuclear pore subcomplex. Indeed, chromatin crosslinking and immunoprecipitation (ChIP) experiments revealed statistically significant increases in the physical interaction between TEL-XI-L and Myc-tagged Nup84, but not Lrs4, upon DSB induction ( Fig. 2a–d ). In addition, the increased interaction between TEL-XI-L and Nup84 was dependent on Lrs4 and Cik1 ( Fig. 2e–g ). Thus, we wondered whether Lrs4 and Cik1 perform mechanistically similar roles at telomeres. However, deletion of Lrs4, but not Cik1, compromised silent chromatin as assessed by ChIP analysis using an antibody specific to histone H3 acetylated at lysines 9 and 14 (diAcH3K9/14), a robust mark of open chromatin ( Supplementary Fig. 2 ) [6] , [8] . Also, unlike Lrs4 deletion, Cik1 loss did not compromise the localization of a green fluorescent protein (GFP)-tagged TEL-XI-L to the nuclear periphery in either the S or G1 phase of the cell cycle ( Fig. 3a–c ). In addition, Nup84 localization to the nuclear periphery was unaffected by the deletion of Lrs4 or Cik1 ( Fig. 3d ). Moreover, cells deficient in the Nup84 component Nup145 exhibited only a very subtle change in perinuclear telomere localization ( Fig. 3a–c ). Together, these findings suggest that cohibin, kinesin-14 and Nup84 complexes may exert different, yet intersecting, functions to promote telomere–Nup84 interactions upon DSB induction. Figure 2: Cohibin and kinesin-14 mediate interaction of subtelomeric DSBs with Nup84. ( a ) Schematic illustrating positions of PCR products used in ChIP to assess interactions between the subtelomeric DSB and various proteins. ( b , c ) Anti-Myc-tagged protein ChIP reveals increased interactions between the subtelomeric DSB and Nup84. Representative gels with ACT1 -normalized relative enrichments ( b ) and quantifications ( c ) are shown (mean±s.d. ; N =3; *, t -test P <0.05). ( d ) Anti-Myc immunoblotting indicates that DSB induction did not alter the level of Myc-tagged proteins used in ChIP analyses. Sir3-Myc served as positive control. ( e , f ) Anti-Myc-tagged protein ChIP also reveals that subtelomeric DSB–Nup84 interactions require Lrs4 and Cik1. Representative gels with ACT1 -normalized relative enrichments ( e ) and quantifications ( f ) are shown (mean±s.d. ; N =3; *, t -test P <0.05). ( g ) Anti-Myc immunoblotting indicates that DSB induction did not alter the level of Myc-tagged proteins used in ChIP analyses. Untag., untagged. 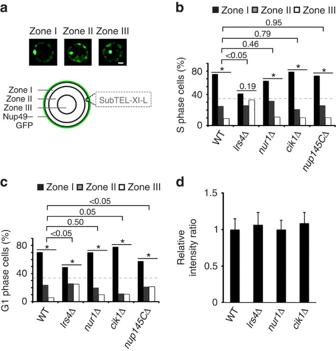Figure 3: Loss of cohibin but not kinesin-14 abrogates perinuclear telomere tethering. (a) Microscopy approach used to assess the position of a GFP-tagged TEL-XI-L relative to the Nup49-GFP-marked nuclear periphery. The tagged telomere can be localized to one of three concentric nuclear zones of equal area. Scale bar, 1 μm. (b,c) Deletion of Lrs4, but not Cik1, strongly abrogates perinuclear telomere positioning during both S phase (b) and G1 phase (c) of the cell cycle. Percentages are presented for the proportion of cells with the telomere located in different nuclear zones (N=100 per genotype). Theχ2testPvalues immediately above bars compare telomere positioning relative to a random (dotted line) distribution (*,χ2testP<0.05). Additional statistical comparisons of cells with different genotypes are as presented. (d) Lrs4 or Cik1 deletion does not affect perinuclear Nup84 localization. Anti-Nup84 immunofluorescence was conducted and the ratio between signal at the nuclear envelope over nucleoplasmic signal was determined; results are presented relative to the wild-type ratio (mean±s.d.;N=10). Full size image Figure 3: Loss of cohibin but not kinesin-14 abrogates perinuclear telomere tethering. ( a ) Microscopy approach used to assess the position of a GFP-tagged TEL-XI-L relative to the Nup49-GFP-marked nuclear periphery. The tagged telomere can be localized to one of three concentric nuclear zones of equal area. Scale bar, 1 μm. ( b , c ) Deletion of Lrs4, but not Cik1, strongly abrogates perinuclear telomere positioning during both S phase ( b ) and G1 phase ( c ) of the cell cycle. Percentages are presented for the proportion of cells with the telomere located in different nuclear zones ( N =100 per genotype). The χ 2 test P values immediately above bars compare telomere positioning relative to a random (dotted line) distribution (*, χ 2 test P <0.05). Additional statistical comparisons of cells with different genotypes are as presented. ( d ) Lrs4 or Cik1 deletion does not affect perinuclear Nup84 localization. Anti-Nup84 immunofluorescence was conducted and the ratio between signal at the nuclear envelope over nucleoplasmic signal was determined; results are presented relative to the wild-type ratio (mean±s.d. ; N =10). Full size image We then asked whether DSB induction promotes kinesin-14 localization to the subtelomeric DSB. Indeed, ChIP analysis revealed that upon DSB induction, there is an Lrs4-dependent increased interaction of Cik1 with the DSB site ( Fig. 4a,b ). These results suggest that cohibin mediates the recruitment of kinesin-14 to the DSB site. This may be achieved by the ability of cohibin to ensure perinuclear telomere anchoring or by a more direct ability of the complex to physically recruit kinesin-14 proteins to the DSB site. However, co-IP experiments failed to detect physical interactions between TAP-tagged Lrs4 and Myc-tagged Nup84 before and after DSB induction ( Fig. 4c ). In contrast, in our positive control cells, interactions between TAP-tagged Heh1 and Myc-tagged Lrs4 were observed in the presence or absence of DSB induction ( Fig. 4c ). Thus, kinesin-14 displays increased localization to the subtelomeric DSB upon its induction in a manner that is likely dependent on cohibin-dependent perinuclear telomere tethering. 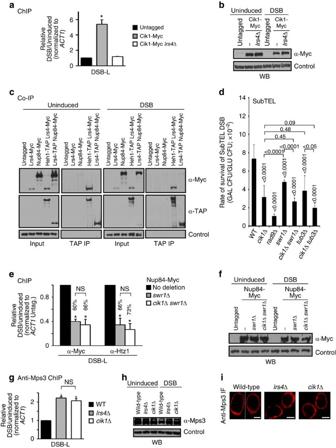Figure 4: Telomeric DSB sensing and preparation for microtubule-dependent repair. (a) Anti-Myc-tagged protein ChIP followed by qPCR analysis reveals Lrs4-dependent increased interactions between the subtelomeric DSB and Cik1 (mean±s.d.;N=2 of triplicates) (*,t-testP≤0.01). (b) Anti-Myc immunoblotting indicates that DSB induction did not alter the level of Myc-tagged proteins used in ChIP analyses. (c) Co-immunoprecipitation using a TAP pull-down reveals no detectable interaction between TAP-tagged Lrs4 and Myc-tagged Nup84. (d) Genetic analysis of subtelomeric DSB repair. Survival (mean±s.d.;N=5) is compiled and presented as the ratio of colony-forming units on galactose (GAL) relative to glucose (GLU).Pvalues (t-test) relative to wild type are presented immediately above mutants. OtherPvalues are as illustrated on the graph. (e) Anti-Myc-tagged Nup84 and anti-Htz1 ChIP followed by qPCR analysis reveals Swr1-dependent chromatin remodelling (mean±s.d.;N=2 of triplicates) (*,t-testP≤0.01). (f) Anti-Myc immunoblotting indicates that DSB induction does not alter the level of Myc-tagged Nup84. (g) Anti-Mps3 ChIP followed by quantitative PCR analysis reveals that induced subtelomeric DSB–Mps3 interactions are increased in cells lacking Lrs4 or Cik1 (mean±s.d.;N=2 of triplicates) (*,t-testP≤0.01). (h) Anti-Mps3 immunoblotting indicates that DSB induction did not alter the level of the protein in our ChIP analysis. (i) Representative immunofluorescence images indicating that the loss of Lrs4 or Cik1 does not alter Mps3 protein localization within the nucleus. Composite images are shown with the scale bar, 2 μm. Untag., untagged. Figure 4: Telomeric DSB sensing and preparation for microtubule-dependent repair. ( a ) Anti-Myc-tagged protein ChIP followed by qPCR analysis reveals Lrs4-dependent increased interactions between the subtelomeric DSB and Cik1 (mean±s.d. ; N =2 of triplicates) (*, t -test P ≤0.01). ( b ) Anti-Myc immunoblotting indicates that DSB induction did not alter the level of Myc-tagged proteins used in ChIP analyses. ( c ) Co-immunoprecipitation using a TAP pull-down reveals no detectable interaction between TAP-tagged Lrs4 and Myc-tagged Nup84. ( d ) Genetic analysis of subtelomeric DSB repair. Survival (mean±s.d. ; N =5) is compiled and presented as the ratio of colony-forming units on galactose (GAL) relative to glucose (GLU). P values ( t -test) relative to wild type are presented immediately above mutants. Other P values are as illustrated on the graph. ( e ) Anti-Myc-tagged Nup84 and anti-Htz1 ChIP followed by qPCR analysis reveals Swr1-dependent chromatin remodelling (mean±s.d. ; N =2 of triplicates) (*, t -test P ≤0.01). ( f ) Anti-Myc immunoblotting indicates that DSB induction does not alter the level of Myc-tagged Nup84. ( g ) Anti-Mps3 ChIP followed by quantitative PCR analysis reveals that induced subtelomeric DSB–Mps3 interactions are increased in cells lacking Lrs4 or Cik1 (mean±s.d. ; N =2 of triplicates) (*, t -test P ≤0.01). ( h ) Anti-Mps3 immunoblotting indicates that DSB induction did not alter the level of the protein in our ChIP analysis. ( i ) Representative immunofluorescence images indicating that the loss of Lrs4 or Cik1 does not alter Mps3 protein localization within the nucleus. Composite images are shown with the scale bar, 2 μm. Untag., untagged. Full size image Next, we asked whether the DNA repair processes studied here intersect with various factors, some of which were previously linked to DSB targeting to the nuclear envelope. For example, the DNA damage response mediator Rad9 (53BP1 in mammals) and Swr1-dependent Htz1 (also known as H2A.Z) incorporation were previously reported to promote DSB mobility [15] . Indeed, we found that subtelomeric DSB repair was greatly dependent on Rad9 ( Fig. 4d ). Survival analysis also revealed that swr1Δ cells had decreased repair efficiency ( Fig. 4d ). Repair was similarly decreased in cik1 Δ and cik1 Δ swr1 Δ cells ( Fig. 4d ). In addition, ChIP analysis indicated that subtelomeric DSB–Nup84 interactions as well as Htz1 incorporation were similarly decreased in swr1 Δ and cik1 Δ swr1 Δ cells ( Fig. 4e,f ). DSBs relocating closer to the nuclear envelope often exhibit increased physical interactions with the Mps3 inner nuclear membrane protein [13] , [15] . Indeed, anti-Mps3 ChIP analysis showed that subtelomeric DSB–Mps3 interaction levels are increased in cells lacking Lrs4 or Cik1 ( Fig. 4g–i ). The similarity between the lrs4 Δ and cik1 Δ cells in these experiments is likely related to the fact that Cik1 displays Lrs4-dependent increased interaction with the induced DSB site ( Fig. 4a,g ). We also assessed DSB repair in cells lacking the α-tubulin subunit Tub3 as a way to destabilize microtubules without inducing severe cellular defects linked to chemical-based microtubule perturbations [44] . Interestingly, tub3 Δ cells displayed decreased DSB repair rates similar to those seen in cik1 Δ cells ( Fig. 4d ). In addition, deletion of Cik1 and Tub3 had a partly additive effect ( Fig. 4d ). These findings suggest that the kinesin-14 complex and microtubules have intersecting yet partly different functions within this DNA repair process. Taken together, these findings provide key mechanistic insights into subtelomeric BIR-dependent DSB repair. Subtelomeric sites experiencing a DSB are subjected to chromatin remodelling and exhibit increased kinesin-14 levels in a manner that is dependent on perinuclear telomere tethering. Such DSBs associate more closely with Mps3 before being ultimately relocated to Nup84 by kinesin-14, which may perform its actions, in part, through cooperation with microtubules. Artificial hyperactivation of subtelomeric DSB repair If targeting the subtelomeric DSB to NPCs is a limiting step in BIR-dependent repair, we would suspect that artificial targeting of the DSB site to NPCs may hyperactivate this DNA repair process. Thus, we integrated near the DSB site on TEL-XI-L either a control DNA sequence or a so-called DNA ‘zip code’ sequence that can artificially target various genetic loci to the NPC ( Fig. 5a ) [45] , [46] , [47] . Spotting assays revealed that the integration of such sequences did not impair the efficiency of DSB induction ( Supplementary Fig. 3 ). ChIP analysis revealed that the zip code sequence, but not the control sequence, led to increased constitutive interaction between the uninduced break site and Nup84 ( Fig. 5b,c ). This was matched with a drastic increase in subtelomeric DSB repair mainly through BIR in wild-type zip code cells as compared with wild-type control sequence cells ( Fig. 5d ). In the absence of Lrs4, Cik1, or control Nup84, the zip code sequence failed to elicit significant increases in constitutive telomere–Nup84 interactions or in subtelomeric DSB repair ( Fig. 5b–d ). The fact that the DNA zip code only increased repair efficiency in wild-type cells but not in cells lacking Lrs4, Cik1 or Nup84, argues against this increased repair being a nonspecific effect related to the zip code disrupting surrounding chromosomal features. In agreement with this rationale, ChIP analysis revealed that the status of diAcH3K9/K14 open chromatin marks near the DSB was similar in cells harbouring zip code and control sequences ( Supplementary Fig. 4 ). These findings strengthen the link between subtelomeric DSB targeting to the NPC and repair efficiency. In addition, these findings indicate that zip codes rely on kinesin-14/Cik1 to relocate DNA within the nucleus. Moreover, failure of the zip code to increase DSB targeting to Nup84 or promote DNA repair in cells lacking Lrs4 can be linked to its role in perinuclear telomere anchoring and/or increased Cik1 recruitment to the induced subtelomeric DSB. 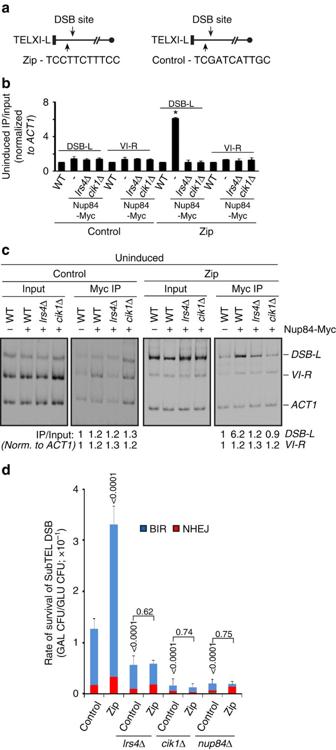Figure 5: Artificial targeting of a subtelomeric DSB to Nup84 hyperactivates BIR. (a) Schematic illustrating the insertion position of the DNA zip or control sequence near the subtelomeric (SubTEL) DSB site. (b) Anti-Myc ChIP reveals that the zip, but not control sequence increases interactions between Myc-tagged Nup84 and the uninduced DSB site, but not control TEL-VI-R. Quantification from three independent experiments are presented (mean±s.d.;N=3; *,t-testP≤0.01). (c) Representative anti-Myc ChIP gel is shown and relative fold enrichments for a region near the subtelomeric DSB site or control TEL-VI-R were calculated for cells harbouring zip or control sequences. Results are normalized toACT1and presented relative to wild-type controls. (d) DSB assay revealing that zip, but not control sequence, hyperactivates BIR-dependent repair in wild type but not cells lacking Lrs4, Cik1 or Nup84 (mean±s.d.,N=5).Pvalues (t-test) comparing control mutants with control wild-type cells are shown immediately above bars. Statistical comparison of zip and control pair are also presented for each of the mutants. Survival analysis was conducted as inFig. 1c,d. Figure 5: Artificial targeting of a subtelomeric DSB to Nup84 hyperactivates BIR. ( a ) Schematic illustrating the insertion position of the DNA zip or control sequence near the subtelomeric (SubTEL) DSB site. ( b ) Anti-Myc ChIP reveals that the zip, but not control sequence increases interactions between Myc-tagged Nup84 and the uninduced DSB site, but not control TEL-VI-R. Quantification from three independent experiments are presented (mean±s.d. ; N =3; *, t -test P ≤0.01). ( c ) Representative anti-Myc ChIP gel is shown and relative fold enrichments for a region near the subtelomeric DSB site or control TEL-VI-R were calculated for cells harbouring zip or control sequences. Results are normalized to ACT1 and presented relative to wild-type controls. ( d ) DSB assay revealing that zip, but not control sequence, hyperactivates BIR-dependent repair in wild type but not cells lacking Lrs4, Cik1 or Nup84 (mean±s.d., N =5). P values ( t -test) comparing control mutants with control wild-type cells are shown immediately above bars. Statistical comparison of zip and control pair are also presented for each of the mutants. Survival analysis was conducted as in Fig. 1c,d . Full size image Kinesin-14 and BIR-dependent repair at non-telomeric loci Next, we asked whether cohibin, kinesin-14 and/or Nup84 are part of a broader BIR process that may be acting beyond telomeres. Therefore, we used a non-telomeric BIR assay in which BIR at an HO-induced break recreates a functional CAN1 gene while removing the HPH hygromycin resistance gene ( Fig. 6a ) [48] . In this system, over 99% of cells surviving the break utilize BIR, which can also be monitored by PCR [48] . Deletion of the BIR factor Pol32 greatly reduced BIR, as expected ( Fig. 6b ). Importantly, disruption of Nup84 or kinesin-14 proteins, but not cohibin, decreased BIR ( Fig. 6b ). BIR kinetics were also impacted in cells lacking Pol32, Cik1 or Kar3 as revealed by PCR analysis ( Fig. 6c ). In addition, Kar3 ATPase domain mutants ( kar3-1 and kar3-898 ) failed to complement kar3 Δ cells and restore full BIR-dependent survival ( Fig. 6d ) [36] , [49] , [50] . kar3-1 and kar3-898 are two Kar3 motor domain mutants that fail to hydrolyse ATP either in general or upon microtubule binding, respectively [49] . This might explain why BIR is slightly higher with kar3-898 as compared with kar3-1 ( Fig. 6d ). Anti-Nup84 ChIP analysis revealed that kar3 Δ cells and kar3-1 cells, respectively, display decreased and increased interaction between the induced DSB site and Nup84 ( Fig. 6e ). We observed this in spite of the fact that both kar3 Δ cells and kar3-1 cells have similarly decreased repair efficiency ( Fig. 6d ). These results suggest that kinesin-14 targets DSBs to and away from Nup84 via mechanistically different processes. This also indicates that both the relocation to and release from Nup84 are important for repair. 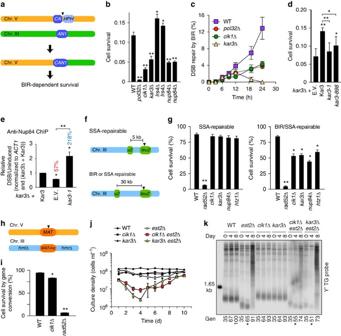Figure 6: Kinesin-14 and Nup84 promote cohibin-independent non-telomeric BIR. (a–d) Roles for kinesin-14 and Nup84, but not cohibin, in non-telomeric BIR. (a) Schematic illustrating galactose-inducible HphMX-marked HO cleavage site (DSB) integrated into theCAN1gene on chromosome (Chr.) V. (b) BIR levels as measured by viability following DSB (mean±s.e.m;N=3; *,t-testP<0.05). (c) The kinetics of BIR as measured by PCR (mean±s.e.m;N=3). (d) Kar3 motor protein ATPase point mutants exhibit compromised BIR-dependent repair (mean±s.e.m;N=3; *,t-testP<0.05). (e) Anti-Nup84 ChIP-quantitative PCR analysis ofkar3Δ cells harbouring plasmid expressing functional Kar3, ATPase point mutantkar3-1, or empty vector (mean±s.d.;N=2 of triplicates; *,t-testP≤0.01). (f,g) Kinesin-14 and Nup84 promote BIR at a DSB site known to localize to the nuclear periphery for repair. (f) Schematic representation of Chr. III DSBs. A galactose-inducible HO endonuclease cleavage site was inserted within theLEU2gene (leu2::cs). One DSB is repairable mainly by SSA, whereas the other can be subjected to SSA or BIR and is targeted to the nuclear periphery during repair13. (g) Quantification of cell survival after DSB induction (mean±s.e.m;N=3; *,t-testP<0.05). (h,i) Cik1 is not required for gene conversion. (h) Schematic illustrating galactose-inducible HO cleavage site (DSB) integrated in the MAT locus on Chr. V in strain lacking donor sequences (HMLandHMR) for homologous recombination but containing aMAT-incregion on Chr. III as donor for gene conversion. (i) Gene conversion efficiency as revealed by cell survival (mean±s.e.m;N=3; *,t-testP<0.05). (j) Spore products ofcik1Δest2Δ andkar3Δest2Δ strains after tetrad dissection showing early accelerated senescence. (mean±s.e.m;N=5). (k) Role for kinesin-14 in telomerase-independent telomere maintenance as revealed by Southern blot indicating thatcik1Δest2Δ cells andkar3Δest2Δ cells exhibit early telomeric defects (*, day 4) relative toest2Δ cells. The number of generations is shown below the blot. Figure 6: Kinesin-14 and Nup84 promote cohibin-independent non-telomeric BIR. ( a – d ) Roles for kinesin-14 and Nup84, but not cohibin, in non-telomeric BIR. ( a ) Schematic illustrating galactose-inducible HphMX-marked HO cleavage site (DSB) integrated into the CAN1 gene on chromosome (Chr.) V. ( b ) BIR levels as measured by viability following DSB (mean±s.e.m; N =3; *, t -test P <0.05). ( c ) The kinetics of BIR as measured by PCR (mean±s.e.m; N =3). ( d ) Kar3 motor protein ATPase point mutants exhibit compromised BIR-dependent repair (mean±s.e.m; N =3; *, t -test P <0.05). ( e ) Anti-Nup84 ChIP-quantitative PCR analysis of kar3 Δ cells harbouring plasmid expressing functional Kar3, ATPase point mutant kar3-1 , or empty vector (mean±s.d. ; N =2 of triplicates; *, t -test P ≤0.01). ( f , g ) Kinesin-14 and Nup84 promote BIR at a DSB site known to localize to the nuclear periphery for repair. ( f ) Schematic representation of Chr. III DSBs. A galactose-inducible HO endonuclease cleavage site was inserted within the LEU2 gene ( leu2::cs ). One DSB is repairable mainly by SSA, whereas the other can be subjected to SSA or BIR and is targeted to the nuclear periphery during repair [13] . ( g ) Quantification of cell survival after DSB induction (mean±s.e.m; N =3; *, t -test P <0.05). ( h , i ) Cik1 is not required for gene conversion. ( h ) Schematic illustrating galactose-inducible HO cleavage site (DSB) integrated in the MAT locus on Chr. V in strain lacking donor sequences ( HML and HMR ) for homologous recombination but containing a MAT-inc region on Chr. III as donor for gene conversion. ( i ) Gene conversion efficiency as revealed by cell survival (mean±s.e.m; N =3; *, t -test P <0.05). ( j ) Spore products of cik1 Δ est2 Δ and kar3 Δ est2 Δ strains after tetrad dissection showing early accelerated senescence. (mean±s.e.m; N =5). ( k ) Role for kinesin-14 in telomerase-independent telomere maintenance as revealed by Southern blot indicating that cik1 Δ est2 Δ cells and kar3 Δ est2 Δ cells exhibit early telomeric defects (*, day 4) relative to est2 Δ cells. The number of generations is shown below the blot. Full size image We also assessed the role of kinesin-14 and Nup84 in the repair of a DSB known to relocate to the nuclear periphery [12] , [13] . We used a system in which Chr. III is modified to harbour an HO-inducible DSB site within a leu2 locus ( Fig. 6f ). Either 5 or 30 kb away from the DSB site, a leu2 segment is also inserted. The 5 kb strain is preferentially repaired by single-strand annealing (SSA) whereas the 30 kb strain undergoes SSA or BIR and is known to relocate to the nuclear periphery for repair ( Fig. 6f ) [13] , [50] . Although the repair of both DSBs were dependent on Rad52, only repair of the 30 kb substrate showed a partial dependency on Cik1–Kar3, Nup84 and Htz1 ( Fig. 6g ). Of note, kinesin-14 was only minimally involved in gene conversion indicating that the observed major impact on BIR systems is not related to unforeseen changes in general DNA donor-based repair processes ( Fig. 6h,i ) [51] . Together, our findings indicate that kinesin-14 and Nup84 are part of a BIR pathway that can act beyond subtelomeric DSBs. We note that although we found kinesin-14 to mediate repair at three of three different BIR-dependent reporter DSB sites tested, it remains unclear if all BIR-dependent repair, or even if BIR-independent repair, implicates kinesin-14 and NPCs. Kinesin-14 maintains telomeres and DSB dynamics BIR is physiologically important for the maintenance of telomeres in the absence of telomerase via a recombination-based mechanism that is akin to the ‘alternative lengthening of telomeres’ seen in telomerase-negative human cancers [39] , [52] , [53] , [54] . Furthermore, eroded telomeres in telomerase-negative yeast cells relocate to nuclear pore complexes, suggesting that the dynamics of telomere localization at the nuclear periphery may be critical for the telomerase-independent maintenance of chromosome ends [23] . To test whether kinesin-14 participates in telomere maintenance in cells lacking the telomerase catalytic subunit Est2, meiotic segregants originating from a common diploid strain were propagated by serial dilution over 10 days and cell densities were recorded daily to estimate cell viability ( Fig. 6j ). Wild-type, cik1 Δ or kar3 Δ cells maintained constant levels of viability over the course of the experiment, whereas est2 Δ cells showed a modest senescence profile manifested by a slight dip in cell viability followed by recovery ( Fig. 6j ). In contrast, the est2 Δ cik1 Δ and est2 Δ kar3 Δ cultures displayed accelerated senescence for 4 days before slowly recovering cell viability by the end of the experiment ( Fig. 6j ). This initial accelerated senescence is reminiscent of telomerase-negative rad52 Δ or pol32 Δ cells, although these latter cells typically fail to exhibit recovery [39] , [52] , [53] . This is consistent with the fact that the loss of Rad52 or Pol32 decreases BIR-dependent repair more drastically than the loss of kinesin-14. More importantly, early accelerated senescence in kinesin-14-deficient est2 Δ cells correlated with a decreased telomeric repeat signal ( Fig. 6k ). Taken together, our findings indicate that kinesin-14 plays a critical role in early telomerase-independent telomere maintenance. We finally tested the possibility that kinesin-14 ensures that damaged DNA maintains a dynamic character, which is needed to move within the nucleus [55] , [56] . Repair of both of our internal and subtelomeric BIR DSB sites is dependent on Rad52 and previous reports using mean square displacement (MSD) analysis revealed that YFP-tagged Rad52 closely follows the dynamics of its DSB sites [55] , [56] . Thus, we examined the dynamics of the induced internal BIR DSB, as well as the subtelomeric DSB sites, in wild-type and kinesin-14-deficient cells. Deletion of Cik1 or Kar3, or expression of the kar3-1 point mutant, in cells harbouring internal BIR DSBs resulted in greatly decreased Rad52–YFP dynamics ( Fig. 7a,b ). Non-damaged DNA moves within the nucleus with a diffusion coefficient D of up to ∼ 10 −3 μm 2 s −1 in yeast, bacteria, flies and mammalian cells [57] . DNA damage would be predicted to increase D beyond this limit. Thus we compared the percentage of cells with D >10 −3 μm 2 s −1 in wild-type and kinesin-14-deficient cells. Deletion of Kar3 or expression of kar3-1, respectively, decreased this percentage from 31.3% in wild-type cells to 4.4 and 11.4% ( Fig. 7b ). In our analysis of Rad52–YFP in the subtelomeric DSB system, Cik1 deletion mildly impacted the MSD curve although a decrease from 21.4 to 14.6% of cells with D >10 −3 μm 2 s −1 was still observed ( Fig. 7c ). This may reflect the fact that, unlike the internal BIR DSB, the subtelomeric DSB is initially closer to the nuclear envelope and so the impact of kinesin-14 on the dynamics of the latter site may be harder to detect. Thus, kinesin-14 allows BIR DSBs to adopt a dynamic character in the nucleus further highlighting the role of DSB mobility in the BIR-mediated repair processes uncovered here. 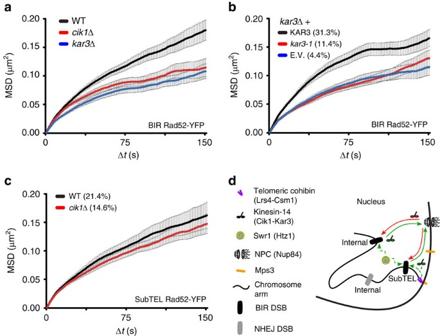Figure 7: Kinesin-14 promotes DSB mobility. (a–c) Mobility of Rad52–YFP foci calculated by mean square displacement (MSD) analysis. Percentage of cells with diffusion coefficientD>10−3μm2s−1is included in parentheses. (a,b) Mobility of non-telomeric BIR-repaired DSBs is shown (N=49). (c) Mobility of subtelomeric (SubTEL) DSBs is shown (N=84). (d) Model depicting BIR-dependent repair processes at subtelomeric and internal DSBs tested. Swr1-dependent Htz1 incorporation allows kinesin-14 to target BIR-repairable DSBs to the nuclear pore subcomplex Nup84 for repair. Cohibin-dependent perinuclear telomere tethering licenses subtelomeric DSBs for this repair process by promoting kinesin-14 recruitment to damaged DNA. DSBs may increase their association with the inner nuclear membrane protein Mps3 along the nuclear envelope before being ultimately targeted to Nup84. DSB targeting to and release from Nup84 via kinesin-14 is performed via non-catalytic and catalytic functions of the complex, respectively. Kinesin-14 performs its role in part via cooperation with microtubules. Dashed arrows symbolize events that promote DSB targeting to the NPC. Green kinesin-14 and arrows highlight DSB targeting to Nup84. Red kinesin-14 and arrows highlight DSB release from Nup84. Figure 7: Kinesin-14 promotes DSB mobility. ( a – c ) Mobility of Rad52–YFP foci calculated by mean square displacement (MSD) analysis. Percentage of cells with diffusion coefficient D >10 −3 μm 2 s −1 is included in parentheses. ( a , b ) Mobility of non-telomeric BIR-repaired DSBs is shown ( N =49). ( c ) Mobility of subtelomeric (SubTEL) DSBs is shown ( N =84). ( d ) Model depicting BIR-dependent repair processes at subtelomeric and internal DSBs tested. Swr1-dependent Htz1 incorporation allows kinesin-14 to target BIR-repairable DSBs to the nuclear pore subcomplex Nup84 for repair. Cohibin-dependent perinuclear telomere tethering licenses subtelomeric DSBs for this repair process by promoting kinesin-14 recruitment to damaged DNA. DSBs may increase their association with the inner nuclear membrane protein Mps3 along the nuclear envelope before being ultimately targeted to Nup84. DSB targeting to and release from Nup84 via kinesin-14 is performed via non-catalytic and catalytic functions of the complex, respectively. Kinesin-14 performs its role in part via cooperation with microtubules. Dashed arrows symbolize events that promote DSB targeting to the NPC. Green kinesin-14 and arrows highlight DSB targeting to Nup84. Red kinesin-14 and arrows highlight DSB release from Nup84. Full size image Our results support a model in which DSBs depend on Swr1/Htz1-dependent chromatin remodelling and kinesin-14 to transiently interact with the nuclear pore subcomplex Nup84 in a BIR-dependent DNA repair pathway ( Fig. 7d ). Perinuclear telomere tethering ensures increased kinesin-14 localization to DSBs thereby licensing them for this broader DNA repair process. Our findings also suggest that DSBs may be targeted to Mps3 before being ultimately relocated in a kinesin-14-dependent manner to Nup84. Kinesin-14 mobilizes DSBs to and away from Nup84 in a manner that is independent and dependent of the catalytic activity of kinesin-14, respectively. These functions of kinesin-14 implicate microtubules. Future work should help clarify how kinesin-14 performs mechanistically different roles to cooperate with microtubules and transiently relocate DSBs to Nup84. It is possible that nuclear microtubule tracks are laid on demand as such structures were recently observed in a different context, quiescence [35] . Cik1–Kar3 is a microtubule minus end-directed motor complex that can only walk on microtubules with a combination of an active (Kar3) and inactive (Cik1) leg [58] . We found that the catalytic activity of Kar3 is required only to release DSBs from Nup84. Thus, it is possible that microtubules are laid with the plus end at NPCs in which case kinesin-14 would have to enlist the catalytic activity of another plus-end-directed motor protein complex to mediate DSB targeting to NPCs. Consistent with this rationale, kinesin-14 type complexes were previously proposed to operate within multi-motor ensembles to collectively organize microtubule networks in vivo [59] , [60] . This arrangement would also be consistent with the fact that microtubule minus ends are relatively static, whereas plus ends are mobile and often engage in so-called dynamic instability, which is defined by cycles of microtubule growth and shortening [61] . DSBs can exhibit greatly increased mobility, which is thought to promote the homology search during recombinational repair [55] , [56] , [62] . These processes may be conserved, as broken DSB ends can exhibit limited or pronounced mobility in mammals [63] , [64] , [65] , [66] . Thus, it will be important to determine whether motor complexes contribute to DSB repair in different organisms including human. We also demonstrate that recently discovered DNA zip codes can be used to target chromosome ends to nuclear pore complexes in a constitutive manner. Interestingly, this action of the zip code is dependent on the telomere-tethering complex cohibin. This may indicate that perinuclear telomere tethering facilitates zip code-dependent targeting of the telomere to NPCs. In contrast, as kinesin-14, unlike cohibin, is not required for perinuclear chromosome tethering, zip code function may directly require the kinesin-14 complex. Taken together, our study supports the notion that DNA zip codes can be used to artificially increase interactions between NPC components and silent chromatin domains such as telomeres. In conclusion, we have uncovered that conserved kinesin-14 and Nup84 proteins cooperate within a BIR pathway that can act on DSBs at different genetic loci. Importantly, BIR-dependent DSB repair is inherently an error-prone process that can compromise overall chromosome integrity. Thus, the herein identified mechanisms may provide DSB survivors with an advantage or disadvantage within a cell population. This may, in turn, be beneficial or deleterious to an organism depending on specific cellular or environmental conditions. Many secondary tumours or resistant cancers emerge from genomic rearrangement in cells exposed to genotoxic therapeutics [67] . It will be important to determine whether error-prone DNA repair processes similar to the one uncovered here play a role in secondary or resistant cancers. In addition, perinuclear telomere tethers have been viewed as guardians of chromosome ends [4] , [21] . However, our findings suggest that in the presence of a DSB, perinuclear tethers can help propagate compromised genomes through engagement of the BIR pathway. Strains and materials Endogenous genes were deleted or modified with C-terminal epitope tags [6] , [8] . Cells were grown to log phase, 5 ml of cell culture was centrifuged, washed with sterile water and resuspended in 100 μl LiOAc mix (100 mM LiOAc pH 7.3, 10 mM Tris-Cl pH 8.0, 1 mM EDTA). Fourteen microlitres of precipitated transformation DNA generated via PCR was added to each sample, followed by the addition of 30 μl salmon sperm single-stranded DNA (10 mg ml −1 ; Invitrogen) and 700 μl PEG (21 g PEG3350, 100 mM LiOAc pH 7.3, 10 mM Tris-Cl pH 8.0, 1 mM EDTA). The transformation mixture was incubated at 30 °C in a water bath for 45 min followed by the addition of 100 μl of DMSO to the sample and then cells were heat shocked in a 42 °C water bath for 15 min. Cells were pelleted via centrifugation and resuspended in 200 μl SOS mix (1 M sorbitol, 1/3v/v YEP media, 6.5 mM CaCl 2 ). Cells transformed with DNA using a drug selection marker was plated onto YEPD media and replica plated the next day onto their respective drug selection plates. Yeast strains are listed in Supplementary Table 3 . Primers for PCR survivor analysis, ChIP and zip code integration are in Supplementary Table 4 . For zip/control sequence integration, primers listed in Supplementary Table 4 and containing either the zip or control sequence were designed and used to amplify a PCR product for transformation following the same protocol used to generate endogenous gene deletions. The NatR cassette gene was used for the selection of integrated strains and the zip/control sequences were ∼ 1.4 kb left of the DSB ( Fig. 5a ). Integration of the zip on the right of the DSB site disrupted DSB induction capacity and so was not used. Chr. XI DSB assays and survivor analysis Strains containing the URA3 cassette flanked by two inverted I-SceI cutting sites at different positions along Chr. XI were transformed by the I-SceI expression plasmid pKM97 (refs 22 , 27 ). This plasmid harbours the I-SceI ORF under control of a galactose-inducible promoter and induction of DSB was performed by plating on galactose media [22] . All subtelomeric ( Figs 1b,c,f,h and 4d ) or internal ( Fig. 1g,h ) DSB survival rates were compiled from at least five platings of two independent pKM97 transformants and compiled wild-type rates are included on the different graphs with t -test statistical analyses comparing either mutant and wild-type strains to each other or indicated mutant strains to each other. A wild-type set was included as an internal reference for every round of mutants plated. For survivor analysis ( Figs 1c and 5d ), at least 30 survivors were analysed by PCR using primer pairs positioned across the DSB site as in Supplementary Table 4 . Survivors identified as BIR were further analysed by PCR using another set of primers (telomeric and more internal on Chr. XI; Fig. 1d ) as presented in Supplementary Table 4 . Non-telomeric BIR assay JRL346-derived strains were grown in XY+2% raffinose before plating onto XY+2% glucose or XY+3% galactose to induce the single DSB [48] . Cells surviving the DSB were replica plated onto Hygromycin B plate to confirm the outcome of repair. The fraction of DSB repair by BIR was calculated by dividing the Hygromycin B sensitive colony-forming units by the initial colony-forming units (cell survival on glucose media). To study the kinetics of BIR, JRL346-derived strains as indicated were grown in XY+2% raffinose and 3% galactose was added in log phase cultures to induce the DSB. Time points were taken at 0, 3, 6, 9, 12, 19 and 24 h post induction and genomic DNA was extracted. Semi-quantitative PCR was used to measure the unique BIR repair product using primers P1 and P2 (ref. 48 ). Gels were imaged using a Bio-Rad Gel Doc XR+ with constant parameters and the resulting images analysed in ImageQuant using volume quantification. Percent repair by BIR was calculated by normalizing the BIR product amplicon signal to the loading control HTA2 amplicon, subtracting the t =0 background signal, and normalizing to genomic DNA from a clone that had undergone BIR. Gene conversion assay Using the TGI354 assay to study ectopic gene conversion, the DSB was induced at the mating type locus (MAT) by galactose-controlled expression of the HO endonuclease [51] . This strain lacks donor sequences (HML and HMR) for homologous recombination. The homologous MAT-inc region on Chr. III is used as a donor for gene conversion. Quantification of cell survival after DSB induction by galactose was then conducted. SSA and BIR assays We used the YMV45 and YMV2 assays to study SSA and BIR in response to DSBs [68] , [69] . The DSB was induced by galactose-controlled expression of the HO endonuclease acting at the cleavage site inside the LEU2 open reading frame ( leu2::cs ) on Chr. III. These cells use a complementary his4::leu2 segment inserted ∼ 5 kb (YMV45) or 30 kb (YMV2) away from the HO cleavage site for DSB repair by SSA (YMV45) or a combination of both SSA and BIR (YMV2). Quantification of cell survival after DSB induction by galactose was then conducted. Spotting assay Cells were spotted starting with 1.25 × 10 5 cells per spot and then in 10-fold serial dilutions onto SC, SC+5FOA or SC-URA media and incubated at 30 °C for 3 days. Cells in which the URA3 reporter is excised by successful galactose-inducible DSB grow on SC+5FOA but not SC-URA media. ChIP For subtelomeric DSB ChIPs, yeast cultures (50 ml) were first grown in SC-leu with 2% raffinose media and then transferred to either SC-leu with 2% glucose (control) or 2% galactose (DSB induction) for 3 h. Cells were similarly treated for non-telomeric DSB ChIPs ( Fig. 6e ) except that SC-trp instead of SC-leu media was used. For uninduced/silencing ChIPs, standard YEPD media was used. In both the cases, cells were grown to a D 600 of 1.8 and cross-linked with 1% formaldehyde at room temperature (RT) for 30 min. The reaction was quenched with glycine at a final concentration of 125 mM for 5 min at RT. Cells were washed with cold TBS (20 mM Tris-HCl pH 7.6 and 150 mM NaCl). Cell pellets were resuspended in 400 μl of lysis buffer (50 mM HEPES-KOH pH 7.5, 500 mM NaCl, 1 mM EDTA, 1% Triton X-100, 0.1% sodium deoxycholate, 0.1% SDS, 1 mM PMSF, 1 tablet of complete protease inhibitor (Roche)). Samples were bead-beated with an equal volume of glass beads 2 × 30 s with intermittent 2 min incubation on ice. Lysates were sonicated 3 × 20 s at 40% amplitude with intermittent incubations on ice. Two consecutive rounds of centrifugation at 16,000 g for 5 and 15 min clarified lysates. One hundred and fifty microlitres of lysate was incubated at 4 °C for 2 h with 2 μg of antibody/sample and further incubated with 15 μl of 50% slurry of pre-washed Protein A-Sepharose beads (GE 17-0870-01) at 4 °C for 1 h. Antibodies used were anti-c-Myc 9E10 (Covance MMS-150R), anti-AcK9/AcK14 H3 (Millipore 06-599), anti-Mps3/Nep98 (gift from Toshiya Endo lab, Nagoya University), anti-Nup84 (Abcam ab122883) and anti-Htz1/H2A.Z (Abcam ab4626). Beads were washed 3 × with lysis buffer, 1 × with LiCl buffer (10 mM Tris-HCl pH 8.0, 250 mM LiCl, 0.5% NP-40, 0.5% sodium deoxycholate, 1 mM EDTA) and 1 × with TE (10 mM Tris-HCl pH 8.0, 1 mM EDTA), and eluted with 50 mM Tris-HCl pH 8.0, 10 mM EDTA and 1% SDS. The eluant was incubated at 65 °C overnight. For Fig. 4a , extra precautionary measures were taken in keeping samples cold because the fusion protein Cik1–Myc13 was particularly sensitive to post-lysis heat-induced degradation. In this case, samples were bead-beated 4 × 15 s and lysates sonicated 6 × 10 s at 40% amplitude with intermittent incubations on ice instead. RNaseA was added at a final concentration of 0.2 μg μl −1 and incubated at 37 °C for 30 min, followed by proteinase K (to 0.2 μg μl −1 ) and glycogen (to 0.03 μg μl −1 ) treatment for 2 h at 37 °C. Dilutions for IP and input DNA were 1:2 and 1:1,000, respectively. PCR parameters were one cycle of 95 °C for 2 min, 55 °C for 30 s and 72 °C for 1 min, followed by 24 to 31 cycles (same within primer sets, optimized for gel analysis) of 95 °C for 30 s, 55 °C for 30 s and 72 °C for 1 min, and a final step of 72 °C for 4 min. Primers and PCR product sizes are listed in Supplementary Table 4 . The PCR products were ethidium bromide (EtBr)-stained. For acrylamide gel-based analyses, relative fold enrichment for the Myc IP reactions is defined as the ratio of the Myc-tagged strains values relative to untagged value according to the following calculation: [DSB IP /ACT1 IP ]/[DSB input /ACT1 input ]. The relative fold enrichments for the anti-diAcH3 reactions were similarly generated. For quantitative PCR analyses, equations taking into account dilution factors and ACT1 control signals were used to calculate enrichments at the given genomic sites. For example, [100 × 2 (adjusted inputsite–Ct (IPsite)) ]/[100 × 2 (adjusted inputACT1–Ct (IPACT1)) ], where adjusted input=CT input −log 2 1,000. Live cell imaging Cells were grown into log phase, pelleted via centrifugation, washed and resuspended in PBS before being mounted onto slides for microscopy. Two-dimensional (2D) images were collected with a Nikon C2+ Confocal Microscope and processed with NIS-Elements AR (Nikon). Using the LacI-GFP fused tetO system, positions of GFP-marked Chr. XI subtelomeres were determined during the S and G 1 phase of the cell cycle with NIS-Elements AR (Nikon) and representative images were adjusted for background using levels and contrast in Photoshop (Adobe). G 1 phase cells were imaged after incubation with 10 μg ml −1 alpha-factor (Sigma) at RT for 3 h. Distance of subtelomeric signal to the nuclear envelope was used to assign localization to one of three concentric nuclear zones of equal area. Immunofluorescence imaging Cells were fixed with 1% formaldehyde, washed and resuspended in SP buffer (1.2 M sorbitol and 0.1 M KH 2 PO 4 pH 7.0). Cells were spheroplasted for 30 min in a digestion mix (40 μg ml −1 lyticase (Sigma) and 0.2% 2-mercaptoethanol in SP buffer) and adhered to diagnostic slides pre-coated with 1 mg ml −1 poly-L-lysine. After blocking in a solution of 1% BSA and 0.1% Triton X-100 in phosphate-buffered saline (PBS) for 1 h, cells were washed with PBS and incubated with goat anti-Nup84 (1:500 in 1% BSA in PBS, Abcam 122883; Fig. 3d ) or rabbit anti-Mps3/Nep98 (1:100 in 1% BSA in PBS, gift from Toshiya Endo lab, Nagoya University; Fig. 4i ) for 1 h at RT. Cells were washed again and incubated with Alexa Fluor 568 rabbit anti-goat (1:750 in 1% BSA in PBS, Life Technologies A11079; Fig. 3d ) or Alexa Fluor 568 goat anti-rabbit (1:500 in 1% BSA in PBS, Life Technologies A11011; Fig. 4i ) for 1 h at RT. Cells were washed and counterstained with 1 μg ml −1 DAPI for 5 min at RT. Samples were washed, Permafluor (Thermo Scientific) was applied as mounting media, and the slides were sealed. The 2D images were collected on a Nikon C2+ Confocal Microscope and processed with NIS-Elements AR (Nikon). The intensity of Nup84 fluorescence at the nuclear periphery and interior was measured with ImageJ (NIH). Whole-cell protein analysis Cells ( D 600 ≈1.0) were subjected to bead-beating with an equal volume of silica beads and lysis buffer (50 mM HEPES-KOH pH 7.5, 150 mM NaCl, 10% glycerol, 0.5% NP-40, 1 mM EDTA, complete tablet protease inhibitor (Roche) and 1 mM PMSF) for 2 × 30 s with an intermittent 2 min incubation on ice. Two consecutive rounds of centrifugation at 16,000 g for 5 and 15 min clarified lysates. Samples were sheared through a 26G½ needle and boiled at 95 °C for 5 min before SDS–PAGE (polyacrylamide gel electrophoresis). Actin immunoblotting served as control. For Figs 2d and 4b , lysates were prepared by the trichloroacetic acid-coupled (TCA) method to eliminate post-lysis protein degradation. For this, 2.5 × 10 7 cells grown to D 600 ≈0.75 were washed and suspended in 500 μl of ice-cold water. Sequential additions of 75 μl of alkali/2-mercaptoethanol (1.85 M NaOH, 1.065 M 2-mercaptoethanol) and 75 μl of 50% trichloroacetic acid solutions were each followed by a 10-min incubation on ice. After centrifugation (9,300 g at 4 °C for 10 min), pellets were suspended in loading buffer (1 × standard loading buffer, 1.42 M 2-mercaptoethanol, 83.2 mM Tris-HCl pH 8.8), boiled and the supernatants were saved [8] . Membranes were probed at 1:1,000 dilutions of HRP-conjugated anti-Myc (Invitrogen R951-25), rabbit anti-Mps3/Nep98 (gift from Toshiya Endo lab, Nagoya University) or mouse anti-Actin (Fisher MA1-744) in TBS with 0.1% Tween-20 and 5% milk. For secondary antibody against Mps3 or actin, HRP-conjugated anti-rabbit IgG (GE NA934) or HRP-conjugated anti-mouse IgG (GE NA931) at 1:2,500 dilution in TBS with 0.1% Tween-20 and 5% milk was used, respectively. All western blots were heavily cropped as a space-saving measure for presentation purposes but full raw images are shown in Supplementary Fig. 5 . CHEF electrophoresis Overnight cell culture (1 ml) was washed and resuspended in 300 μl of EDTA/Tris (50 mM EDTA, 10 mM Tris-HCl pH 7.5). Zymolyase (2 μl of 20 μl ml −1 in 10 mM Na 2 HPO 4 pH 7.5) and 500 ml of low melting-point CHEF-quality agarose (1% in 125 mM EDTA pH 8.0, 42 °C) were added and the mixture was solidified in plug moulds at 4 °C. Plugs were incubated overnight in 1 ml of 10 mM Tris-HCl pH 7.5, 500 mM EDTA at 37 °C, then overnight in 1 ml of 2 mg ml −1 proteinase K in 10 mM Tris-HCl pH 7.5, 500 mM EDTA, 10 mg ml −1 N-lauroylsarcosine at 50 °C. Plugs were washed three times with EDTA/Tris (4 °C, 1 h per wash) and stored in 2 ml of EDTA/Tris (4 °C). Plugs and ladder (standard S. cerevisiae ; Bio-Rad) were cut to 5 mm × 3 mm × 1.5 mm and resolved (24 h, 6.0 V cm −1 , 45–95 s, 14 °C) on a 0.8% CHEF agarose gel in 0.5 × TBE using the CHEF-DR-II apparatus (Bio-Rad). Gels were EtBr-stained and imaged. Co-immunoprecipitation Yeast cultures (50 ml) were first grown in SC-leu with 2% raffinose media and then transferred to either SC-leu with 2% glucose (control) or 2% galactose (DSB induction) for 3 h until D 600 ∼ 1.6 and normalized to 5 × 10 7 cells. Cells were washed with 50 mM Tris-HCl pH 7.5 and 150 mM NaCl. Cells were bead-beated with 400 μl of lysis buffer (50 mM HEPES-KOH pH 7.5, 150 mM NaCl, 10% glycerol, 0.5% NP-40, 1 mM EDTA, 1 mM PMSF and one tablet of complete protease inhibitor (Roche)) and glass beads 2 × 30 s with intermittent 2 min incubation on ice. Clarified extracts were incubated with 30 μl of a 50% slurry of pre-washed IgG Sepharose beads (GE) for 2 h at 4 °C. Beads were washed with 1 ml of lysis buffer six times. In all, 5% of input whole-cell extract and 25% of Lrs4-TAP- or Heh1-TAP-bound fractions were run on 8% SDS–PAGE gels. Membranes were probed at 1:1,000 dilutions of HRP-conjugated anti-Myc (Invitrogen R951-25), HRP-conjugated anti-TAP (Sigma P1291) or mouse anti-Actin (Fisher MA1-744) in TBS with 0.1% Tween-20 and 5% milk. For secondary antibody against actin, HRP-conjugated anti-mouse IgG (GE NA931) at 1:2,500 dilution in TBS with 0.1% Tween-20 and 5% milk was used. Mobility analysis Yeast expressing Nup49–mCherry and Rad52–YFP were grown in SD-leu supplemented with 2% raffinose overnight to 2.5–5 × 10 6 cells ml −1 with additional selection for plasmids as required. Galactose was added for 2.5 h to induce a DSB at 3% final concentration. Cell were mounted in a concanavalin A-coated eight-well chamber (LabTek II, Nalge-Nunc) and maintained at 30 °C. Live cell time-lapse microscopy was performed using a DeltaVision Elite (Applied Precision) with a × 100/1.40 NA plan Apochromat oil immersion objective (Olympus) and CoolSNAP HQ2 CCD Camera (512 × 512 with 2 × 2 bin, Roper Scientific). Single plane images were acquired in the YFP channel every 1.5 s for 180 s (490 nm excitation, 200 ms exposure) while mCherry images were captured every fifth frame (575 nm excitation, 200 ms exposure). Nuclear alignment was performed using Nup49–mCherry frames with a custom MATLAB script while Rad52–YFP was tracked using the SpotTracker plugin in ImageJ to yield x , y coordinates [70] . Final MSD analysis was calculated using a custom MATLAB script. We used the slope ( m ) of the first five time intervals (1.5–7.5 s) to determine the 2D diffusion coefficient ( D ) given that D = m /2 × d , where d is the number of dimensions. The radius of confinement was calculated as Rc =5/4 × √MSD calculated from the average MSD value of the last 20 time intervals (121.1–150 s). Telomerase-independent senescence Cells were grown to saturation in 10 ml cultures of XY with 2% glucose and diluted to 5 × 10 5 cells ml −1 every 24 h. Cell density was measured using a hemocytometer. Samples were taken at days 0, 4 and 8 for telomere length analysis by Southern blotting. Genomic DNA was digested with XhoI and probed with a Y’-TG probe generated from the pYT14 plasmid [1] . The approximate number of generations was calculated on the basis of the initial growth on plates after sporulation (3 days) and the cell density during liquid culturing. How to cite this article: Chung, D. K. C. et al . Perinuclear tethers license telomeric DSBs for a broad kinesin- and NPC-dependent DNA repair process. Nat. Commun. 6:7742 doi: 10.1038/ncomms8742 (2015).